Melt migration in basalt columns driven by crystallization-induced pressure gradients The structure of columnar-jointed lava flows and intrusions has fascinated people for centuries and numerous hypotheses on the mechanisms of formation of columnar jointing have been proposed. In cross-section, weakly developed semicircular internal structures are a near ubiquitous feature of basalt columns. Here we propose a melt-migration model, driven by crystallization and a coeval specific volume decrease inside cooling and solidifying columns, which can explain the observed macroscopic features in columnar-jointed basalts. We study basalts from Hrepphólar (Iceland), combining macroscopic observations, detailed petrography, thermodynamic and rheological modelling of crystallization sequences, and Anisotropy of Magnetic Susceptibility (AMS) of late crystallizing phases (that is, titanomagnetite). These are all consistent with our proposed model, which also suggests that melt-migration features are more likely to develop in certain evolved basaltic lava flows (with early saturation of titanomagnetite), and that the redistribution of melt within individual columns can modify cooling processes. Columnar jointing is a common feature in many basaltic lava flows and intrusions around the world. Spectacular arrangements of columns have fascinated observers for centuries, and numerous hypotheses on their origin have been proposed [1] , [2] , [3] , [4] , [5] , [6] , [7] , [8] , [9] . Diffuse semi-circular structures occurring inside basalt columns have previously been described by several authors [5] , [7] , with suggestions that these internal features could be formed by constitutional supercooling [4] , [5] . However, constitutional supercooling (generating interface instabilities between melt and solids) alone cannot fully explain either the development of columnar jointing [5] or the observed internal structures. An alternative model explains viscous fingering inside columns as a result of a double-diffusive convective process, with this viscous fingering being the underlying cause for the formation of columnar jointing [7] . This hypothesis is also in sharp contrast to many field observations where column-delimiting fractures frequently cross-cut the internal textures [5] which they clearly must post-date. To better understand the formation of these enigmatic internal features formed during crystallization of basaltic melts, a combined textural, geochemical and physical modelling approach is required. Columnar-jointed basalts from Hrepphólar (Iceland) display strong evidence for internal melt migration parallel to the column axis. Here we present a simple physical model, driven by gravity and decrease of the specific volume during crystallization, which explains the formation of the internal structures. In response to progressive cooling, and increased load of overlying material, a pressure-gradient develops near the base of the columns which drives melt migration into the columns. This hypothesis, supported by petrographic observations, physical modelling and by the variation in the anisotropy of magnetic susceptibility (AMS) across a basalt column, offers a viable mechanism to redistribute melt into the individual columns. We suggest that this process is not unique to Hrepphólar but is likely to occur during solidification of most thick lava flows that develop columnar jointing. Petrographic textures and field observations Basalt columns in a thick lava flow from Hrepphólar (Iceland) display striking internal structures when polished. Alternating diffuse dark and light bands result from variable modal proportions of the main phenocryst phases (that is, plagioclase, clinopyroxene, olivine and titanomagnetite). Thin sections from a profile across a column show typical seriate texture and discontinuous plagioclase chains ( Fig. 1 ). Similar plagioclase chains have previously been described in detail from other thick, slowly solidifying, lava flows [10] , [11] . When cut parallel to the column axis ( Fig. 2a ), the polished surfaces of the Hrepphólar columns reveal evidence of viscous fingering, implying vertical movement of melt within the column ( Fig. 2b,c ). In cross-section ( Fig. 2d ), banding near the edge of the column forms pseudo-hexagonal shapes that successively become more rounded towards the centre ( Fig. 2e,f ). Approximately 20% of this pseudo-hexagonal banding is cross-cut by the column-bounding joints ( Fig. 2f ) and must thus have formed prior to the jointing. 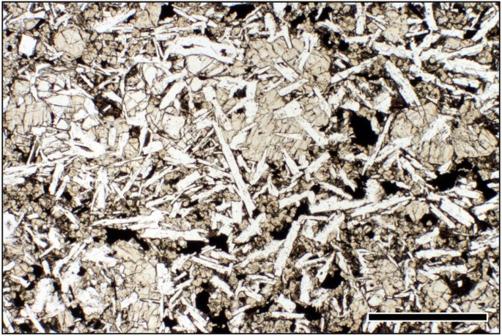Figure 1: Plagioclase chains in the Hrepphólar columns. Thin section image (plane-polarized light) showing the main petrographic textures of basalt from Hrepphólar (Iceland). Note the distinct linking of plagioclase laths (bright white) into framework-forming chains. The groundmass between plagioclase chains is dominated by clinopyroxene (light brown) and titanomagnetite (black). The scale bar is 10 mm and the vertical axis of the image is orientated parallel to the section's original orientation (vertical, and the right way up). Figure 1: Plagioclase chains in the Hrepphólar columns. Thin section image (plane-polarized light) showing the main petrographic textures of basalt from Hrepphólar (Iceland). Note the distinct linking of plagioclase laths (bright white) into framework-forming chains. The groundmass between plagioclase chains is dominated by clinopyroxene (light brown) and titanomagnetite (black). The scale bar is 10 mm and the vertical axis of the image is orientated parallel to the section's original orientation (vertical, and the right way up). 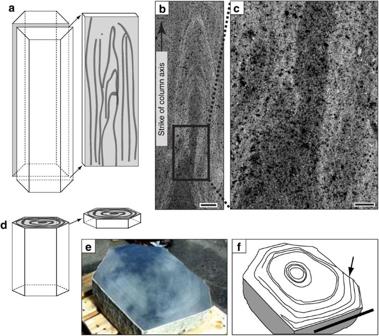Figure 2: Internal structures in columnar-jointed basalt from Hrepphólar. (a) Schematic illustration of a vertical cross-section through a column. (b) Polished cross-section along the main axis of the column. Scale bar is 15 mm. (c) Magnification of the same plate showing viscous fingering in the central part of the column. Scale bar is 5 mm. (d) Schematic illustration of a horizontal cross-section through a column. (e) Polished cross-section cut perpendicular to the column axis. (f) Schematic illustration of the same sample with banding. Scale bar is 52 cm. Note that several of the internal structures are cut by the column-bounding fracture (indicated by arrow in (f)). Also note that for clarity the photographs in (b) and (c) are inverted (dark areas in the photograph correspond to brighter areas in the natural sample and vice versa). See alsoSupplementary Figures S1, S2, S3for more examples. Full size image Figure 2: Internal structures in columnar-jointed basalt from Hrepphólar. ( a ) Schematic illustration of a vertical cross-section through a column. ( b ) Polished cross-section along the main axis of the column. Scale bar is 15 mm. ( c ) Magnification of the same plate showing viscous fingering in the central part of the column. Scale bar is 5 mm. ( d ) Schematic illustration of a horizontal cross-section through a column. ( e ) Polished cross-section cut perpendicular to the column axis. ( f ) Schematic illustration of the same sample with banding. Scale bar is 52 cm. Note that several of the internal structures are cut by the column-bounding fracture (indicated by arrow in ( f )). Also note that for clarity the photographs in ( b ) and ( c ) are inverted (dark areas in the photograph correspond to brighter areas in the natural sample and vice versa). See also Supplementary Figures S1, S2, S3 for more examples. Full size image To characterize the observed internal textures and develop a conceptual model for their formation we produced a polished plate (300×700×10 mm), cut as a traverse through the central parts of a column (where the flow features are most prominent; see Fig. 2a,b ). Thermodynamic and rheological modelling of the solidification process From a representative composition of the Hrepphólar basalt ( Supplementary Table S1 ) equilibrium crystallization and mineral reactions were calculated between 1,150 and 975 °C ( Fig. 3a ). Density changes over the explored temperature interval occur due to both the thermal expansivity of each phase and the continually evolving mineral–melt proportions and compositions. Following the initiation of plagioclase crystallization at ca. 1,150 °C, calculated system density (melt and crystal densities combined proportionally) increases from approximately 2750 kg m −3 to >3200 kg m −3 at the solidus ( Fig. 3b ). The specific volume thus decreases by more than 15% over this interval. Calculations also suggest resorption of early olivine during cooling, primarily forming Ca-poor pigeonite (which coexists with Ca-rich augite). A small fraction of olivine crystals are, however, present in the Hrepphólar columns ( ≪ 10 modal%). We interpret this as recording a key difference between thermodynamic and natural systems, with the latter requiring sufficiently slow cooling to overcome kinetic barriers for the reaction. We emphasize, however, that this minor deviation in final assemblage has little impact on subsequent results because the modal volume of the respective phases (olivine and Ca-poor clinopyroxene) is low and their densities similar. Predicted early and late augite compositions match well with core and rim compositions of analysed clinopyroxene crystals. 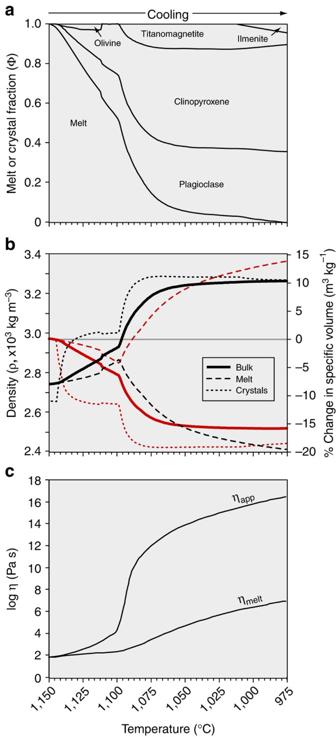Figure 3: Thermodynamic and rheological modelling of the Hrepphólar system. (a) Fractions of each crystallizing phenocryst phase and the remaining melt as a function of temperature. (b) Density and specific volume change (relative to 1,150 °C) of the system (bulk), and crystal and melt fractions. Black lines represent density changes and red lines specific volume change. (c) Calculated melt viscosity (ηmelt) and modelled apparent viscosity (ηapp) based on the predicted crystal content at each temperature. Note that the modelling covers the temperature interval 1,150 °C to 975 °C (see alsoSupplementary Data 1and2for modelled phase proportions and melt composition). Also note that there is a drastic change in the melt/crystal densities and the apparent viscosity (melt+crystals) corresponding to the saturation of titanomagnetite (at approximately 1,100 °C). Figure 3: Thermodynamic and rheological modelling of the Hrepphólar system. ( a ) Fractions of each crystallizing phenocryst phase and the remaining melt as a function of temperature. ( b ) Density and specific volume change (relative to 1,150 °C) of the system (bulk), and crystal and melt fractions. Black lines represent density changes and red lines specific volume change. ( c ) Calculated melt viscosity (η melt ) and modelled apparent viscosity (η app ) based on the predicted crystal content at each temperature. Note that the modelling covers the temperature interval 1,150 °C to 975 °C (see also Supplementary Data 1 and 2 for modelled phase proportions and melt composition). Also note that there is a drastic change in the melt/crystal densities and the apparent viscosity (melt+crystals) corresponding to the saturation of titanomagnetite (at approximately 1,100 °C). Full size image The evolving melt compositions calculated above ( Fig. 3a and Supplementary Data 1 , 2 ) were used to calculate viscosities with the equations of refs 12 , 13 . For crystal fractions less than 0.4 (that is, T > 1,100 °C) there is no significant viscosity contrast between melt and the bulk system ( Fig. 3c ). However, at approximately 1,090 °C, shortly after the onset of titanomagnetite crystallization, the melt density drops rapidly ( Fig. 3b ) in response to the change in chemistry as the apparent (melt+crystals) viscosity of the system increases dramatically ( Fig. 3c ). Previous modelling of the density change associated with solidification of the Holyoke flood basalt [14] (with a Fe/Mg ratio of 2.0, compared with 2.5 in Hrepphólar) yielded a net change in specific volume of −12% in the interval 0–91% crystals, 1,200–800°C. Although this flow represents a significantly different composition and Mg/Fe ratio to that used for our calculations, a large decrease in specific volume is still predicted. This implies that the total magnitude of the volume change associated with solidification of basaltic lavas is not strongly sensitive to the melt composition. However, we note that there is a tendency for more evolved basalts (Fe-rich) to saturate titanomagnetite earlier in the crystallization sequence, affecting the solid density and thus leading to a slightly larger decrease in specific volume. In a lava flow, the ∼ 15% volume decrease predicted by the thermodynamic modelling, above, must affect the body equally in its vertical and horizontal components. The vertical component may be explained by simple contraction or compaction [10] , [11] , [14] , [15] , whereas the lateral component can only partly be explained by the spacing between individual columns. This free-space typically measures <2 mm, forming column-delimiting joints between 1 m-diameter columns (that is, <0.5%). A significant portion of the lateral component thus remains unaccounted for. Measurements of anisotropy of magnetic susceptibility (AMS) If the banding observed in the Hrepphólar columns results from melt-migration processes, this should also be reflected by internal textures (for example, mineral orientations). Elongated plagioclase crystals can show preferential orientation in an applied stress-field (that is, in response to flow). However, as plagioclase can become locked in a 3-dimensional network early in the crystallization history [11] , it is desirable here to use an alternative indicator for direction. A late crystallizing phase, such as titanomagnetite, should better retain information on flow conditions during the last stages of crystallization. Therefore, we measured the anisotropy of magnetic susceptibility (AMS) [16] on 27 cubic (1 cm 3 ) samples across a single column ( Fig. 4 ). Results are represented by an ellipsoid with principal axes of susceptibility, k 1 ⩾ k 2 ⩾ k 3 . Previous AMS-studies aimed at determining flow directions in columnar-jointed basalts have generated inconclusive results with respect to observed macrofabrics [6] , [17] , [18] , [19] , [20] , [21] , [22] , [23] . In contrast to previous studies we measured the AMS with a high-field torsion magnetometer, which is insensitive to magnetic domain state and allows separate determination of paramagnetic and ferrimagnetic ( sensu stricto ) sub-fabrics [24] ( Fig. 4 ). The paramagnetic sub-fabric (clinopyroxene and olivine) shows a broader dispersion compared with the ferrimagnetic sub-fabric (titanomagnetite). This is related partly to the intrinsic anisotropy of these minerals but also to the fact that clinopyroxene and olivine begin to crystallize at a relatively early stage, with clinopyroxene continuing to crystallize over a broad temperature interval (1,141–975°C). These minerals may therefore be locked in position by the early crystallizing network of plagioclase chains and develop little preferred orientation. Titanomagnetite, on the other hand, crystallizes late (<1,100 °C) and its AMS is controlled by shape in the case of non-euhedral crystals. Here the k 1 -axes cluster very close to the long axis of the basalt column ( Fig. 4 ). We interpret this as reflecting an alignment of titanomagnetite crystal long-axes imparted by melt migration. 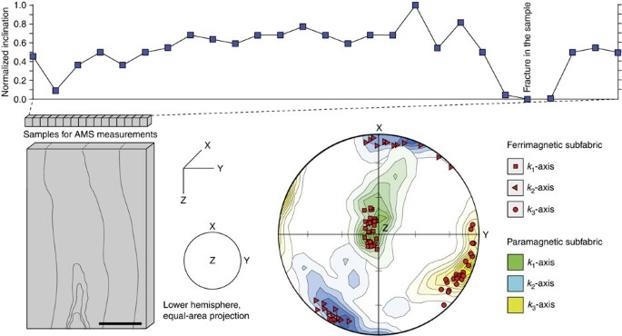Figure 4: AMS measurements across a basalt column. The top figure shows inclination of the k1-axis of titanomagnetite across a horizontal profile through the basalt column. Note that the inclination (normalized between 67° and 88°) systematically increases towards the centre of the plate approaching near vertical orientations in the centre. AMS data are plotted in the stereographic projection with respect to the coordinate system used to describe the basalt plate. Scale bar on the schematic illustration of the plate is 10 cm. Specimens were sampled from the top of the plate, and across the plate. For the ferrimagnetic (paramagnetic) anisotropy, squares (green shading) are axes of maximum susceptibility, triangles (blue shading) are axes of intermediate susceptibility, and circles (yellow shading) are axes of minimum susceptibility. Each contour represents an increase of two standard deviations (that is, ɛ, 2σ, 4σ, 6σ, ...), compared with the expected standard deviation for a uniform distribution of data (based on the same number of data records). Note that each principal axis was contoured individually. Contour intervals were computed using a Gaussian counting method, with the Spheristat software (Pangea Scientific). Figure 4: AMS measurements across a basalt column. The top figure shows inclination of the k 1 -axis of titanomagnetite across a horizontal profile through the basalt column. Note that the inclination (normalized between 67° and 88°) systematically increases towards the centre of the plate approaching near vertical orientations in the centre. AMS data are plotted in the stereographic projection with respect to the coordinate system used to describe the basalt plate. Scale bar on the schematic illustration of the plate is 10 cm. Specimens were sampled from the top of the plate, and across the plate. For the ferrimagnetic (paramagnetic) anisotropy, squares (green shading) are axes of maximum susceptibility, triangles (blue shading) are axes of intermediate susceptibility, and circles (yellow shading) are axes of minimum susceptibility. Each contour represents an increase of two standard deviations (that is, ɛ, 2σ, 4σ, 6σ, ...), compared with the expected standard deviation for a uniform distribution of data (based on the same number of data records). Note that each principal axis was contoured individually. Contour intervals were computed using a Gaussian counting method, with the Spheristat software (Pangea Scientific). Full size image We also note that there is a clear systematic variation in the inclination of the k 1 -axis in titanomagnetite across the plate ( Fig. 4 ), with the steepest inclinations measured in the central parts (dipping at 88°). Although, a later fracture affects the symmetry across the measured plate the inclinations of titanomagnetite follow the general geometry of the observed banding ( Fig. 2 ). Cooling of thick lava flows has been shown to be dominated by conductive heat loss [25] , [26] . This occurs simultaneously from the top and base of the lava flow [25] , [26] , [27] and to the column-bounding fractures. Cracks propagate with cooling, resulting in an inhomogeneous temperature distribution within each column. Isotherms below the crack propagation front will be aligned sub-horizontally ( Fig. 5a ) and controlled by conductive heat loss to the upper surface of the lava flow [3] . As fractures continue to propagate to depth, heat loss to the sides of the columns becomes more important. Because at depth, the distance to a fracture is substantially shorter than that to the outer surface of the lava flow [3] , the resultant isotherms gradually steepen with time, eventually becoming sub-vertical in parts of the column ( Fig. 5b ). Any water present in the fractures during solidification significantly increases the cooling rate [28] , resulting in even steeper isotherms. An important consequence of this isotherm steepening is that strongly heterogeneous thermal, textural and rheological structures form at any particular depth, with rapid cooling of the column walls. 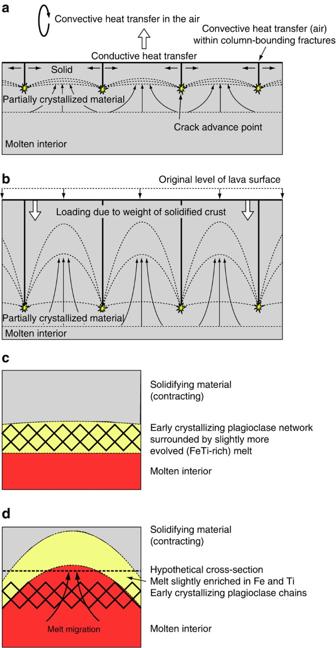Figure 5: Cooling, solidification and development of the melt migration structures. Schematic illustration of progressive cooling and change in orientation of isotherms within a thick, columnar-jointed, lava flow due to conductive cooling to the top and sides of individual columns (modified from ref.3). (a) Early in the cooling history column-bounding cracks are shallow and do not significantly affect the orientation of individual isotherms. (b) As the crack propagation front penetrates deeper into the lava flow, cooling from the top becomes less important than that from the sides. This results in steepening of isotherms. (c) Schematic sketch showing the interface between melt and partially crystallized material. Plagioclase chains are first to crystallize (Fig. 3a) and join together to form networks along sub-horizontal isotherms. The melt immediately surrounding the plagioclase chains becomes enriched with respect to Fe and Ti compared with its original composition. (d) Continuous cooling in combination with increased loading from the solidified crust creates an internal pressure gradient which migrates melt upward to accommodate the volume-loss associated with crystallization. Note that this process involves slight variations in melt composition, which are also necessary for producing the viscous fingering structures depicted inFig. 2b,c. Figure 5: Cooling, solidification and development of the melt migration structures. Schematic illustration of progressive cooling and change in orientation of isotherms within a thick, columnar-jointed, lava flow due to conductive cooling to the top and sides of individual columns (modified from ref. 3 ). ( a ) Early in the cooling history column-bounding cracks are shallow and do not significantly affect the orientation of individual isotherms. ( b ) As the crack propagation front penetrates deeper into the lava flow, cooling from the top becomes less important than that from the sides. This results in steepening of isotherms. ( c ) Schematic sketch showing the interface between melt and partially crystallized material. Plagioclase chains are first to crystallize ( Fig. 3a ) and join together to form networks along sub-horizontal isotherms. The melt immediately surrounding the plagioclase chains becomes enriched with respect to Fe and Ti compared with its original composition. ( d ) Continuous cooling in combination with increased loading from the solidified crust creates an internal pressure gradient which migrates melt upward to accommodate the volume-loss associated with crystallization. Note that this process involves slight variations in melt composition, which are also necessary for producing the viscous fingering structures depicted in Fig. 2b,c . Full size image The increased load imposed by the solidified crust, in combination with the stresses associated with volume loss inside the column, drives melt migration from the base to the interior of the columns, roughly following the isotherms ( Fig. 5 ). The main source of melt is located close to the interface of molten and partially crystallized layers ( Fig. 5 ). Here it is important to emphasize that melts having experienced variable crystallization (depending upon their position in the thermal structure) are involved in the migration process at Hrepphólar. In particular, melt, from which the plagioclase network crystallized (enriched in Fe and Ti relative to the original composition), can be juxtaposed with less-evolved melts from the interior of the lava flow ( Fig. 5c,d ). During solidification these develop a contrasting, banded appearance (that is, the dark and light bands have 7 and 4 modal% titanomagnetite, respectively). The viscous fingering ( Fig. 2b,c ) also provides compelling evidence for local variations in the melt composition. Although melt migration is intimately associated with the propagation of column-bounding fractures, it must predate cracking at any structural depth, as shown by the cross-cutting relations ( Fig. 2f ). Convection, due to internal temperature contrasts, can potentially produce structures similar to those observed at Hrepphólar. However, significant convection within individual columns at Hrepphólar can be ruled out for two reasons: the elongated geometry of individual columns are unfavourable for maintained convection of molten material [2] , and Hrepphólar exhibits evidence for unidirectional (upwards) migration within the columns but lacks reverse (downwarping) features, typically produced by convection. The following crystallization scenario for the Hrepphólar columns is envisaged. First, plagioclase chains begin to form ( Figs 1 and 3a ), locking together into a 3-dimensional network near the interface between molten and partially crystallized material ( Fig. 5c ). Previous studies have confirmed that this occurs early in the crystallization history, at melt proportions as high as 75% (ref. 10 ). This plagioclase network is strong, and resists much of the deformation associated with melt migration. However, such networks are also permeable [10] allowing continuous migration of melt through the network. Thermodynamic modelling of the Hrepphólar system suggests that when a crystal fraction of ∼ 0.5 is reached, the residual melt density drops significantly ( Fig. 3b ). The apparent viscosity of the system sharply increases at this point, whereas the melt viscosity only marginally increases. Combined, these factors indicate that it is far easier to move liquid through the partially crystallized framework of plagioclase chains than deforming the framework itself. The mobility of this liquid is strongly influenced by the saturation of titanomagnetite, which rapidly lowers the melt density. The presence of modal layering is the main factor that allows us to observe melt migration in the Hrepphólar columns. This suggests that evidence for melt migration should be most prominent in thick lava flows which cool slowly and form wide columns. Thinner and more rapidly cooled lava flows do not have sufficient time to develop the clear geochemical differences necessary to record such migration (although late-crystallizing phases may still be aligned). This strongly implies that the process of melt migration is not unique to Hrepphólar, but may be a common phenomenon in many thick basaltic lava flows that developed columnar jointing. Indeed, similar internal structures have been briefly described from various other locations [5] (see also Supplementary Figs S1, S2, S3 ), although there is currently no comprehensive study characterizing internal variations within individual columns. It is likely that geochemical variation within a single column will be minor because of the near-continuous mix of early crystallizing compositions (plagioclase chains trapping clinopyroxene) with late-crystallizing phases including titanomagnetite, plagioclase and clinopyroxene. A far more direct method for constraining melt migration during the last stages of crystallization comes from AMS-measurements of titanomagnetite. The process of melt migration proposed here has implications for our understanding of both the petrological and thermal evolution of columnar-jointed lava flows. For example, simple static conductive cooling models commonly used to explain the solidification of basaltic lava flows may be inappropriate as temperature and physical properties change in response to the melt migration within individual columns. We believe that further investigations of the compositional control on the development on melt-migration features is necessary to understand, and potentially also predict, the cooling processes of chemically diverse lava flows. Thus, focused research on the processes associated with the formation and evolution of columnar-jointed lavas and intrusions may continue to yield important information on the mechanical, thermal and petrological conditions experienced during magma solidification. Thermodynamic modelling We quantified mineral–melt equilibria associated with cooling and crystallization in the basaltic system using the MELTS program and thermodynamic data [29] , [30] . Pressure was fixed at 10 bars (representing approximately 30 m depth in the Hrepphólar lava flow). Equilibrium crystallization and mineral reactions were calculated, assuming a closed system with a fixed initial Fe 2+ /Fe 3+ ratio and no imposed constraint of the oxygen fugacity (see Supplementary Data 1 and 2 for the modelled basalt composition). f O 2 subsequently varied over the temperature interval 1,150 to 975 °C from QFM -1.22 to QFM -0.70. AMS measurements Bulk susceptibility and low-field AMS were measured using an AGICO KLY-2 Kappabridge. AMS measurements were performed with a standard 15 position measurement scheme [31] , from which it is possible to determine the complete symmetric second-rank susceptibility tensor. The eigenvectors and eigenvalues of the tensor represent the orientation and magnitude of the three principal susceptibility axes, k 1 ⩾ k 2 ⩾ k 3 , which is represented geometrically by an ellipsoid. Additionally, a high-field torque magnetometer was used for AMS measurements [32] , using 7 different applied fields ranging from 700 to 1500 mT. The magnetic torque was corrected with respect to the specimen holder signal and zero applied field, the latter correcting the magnetic torque signal in the absence of an applied field. Torque measurements provide the deviatoric susceptibility, which expresses the anisotropy in terms of the deviation from a sphere, with principal axes l 1 ⩾ l 2 ⩾ l 3 , where l 3 is always negative and l 2 can be either positive or negative depending on the shape of the susceptibility ellipsoid. Separation of the AMS due to paramagnetic and ferrimagnetic ( s.s. ) minerals was done using the procedure of ref. 24 . How to cite this article: Mattsson, H.B. et al . Melt migration in basalt columns driven by crystallization-induced pressure gradients. Nat. Commun. 2:299 doi: 10.1038/ncomms1298 (2011).